NMR structure of human restriction factor APOBEC3A reveals substrate binding and enzyme specificity Human APOBEC3A is a single-stranded DNA cytidine deaminase that restricts viral pathogens and endogenous retrotransposons, and has a role in the innate immune response. Furthermore, its potential to act as a genomic DNA mutator has implications for a role in carcinogenesis. A deeper understanding of APOBEC3A’s deaminase and nucleic acid-binding properties, which is central to its biological activities, has been limited by the lack of structural information. Here we report the nuclear magnetic resonance solution structure of APOBEC3A and show that the critical interface for interaction with single-stranded DNA substrates includes residues extending beyond the catalytic centre. Importantly, by monitoring deaminase activity in real time, we find that A3A displays similar catalytic activity on APOBEC3A-specific TT C A- or A3G-specific CC C A-containing substrates, involving key determinants immediately 5′ of the reactive C. Our results afford novel mechanistic insights into APOBEC3A-mediated deamination and provide the structural basis for further molecular studies. The human APOBEC3 (A3) proteins are a family of deoxycytidine deaminases that convert dC residues in single-stranded DNA (ssDNA) to dU, and act as DNA mutators. These proteins, which have an important role in the innate immune response, function as host restriction factors and display a broad range of activities against endogenous and exogenous retroelements [1] , [2] , [3] . There are seven members in the A3 family, each having one (A3A, A3C, A3H) or two (A3B, A3D, A3F, A3G) zinc (Zn)-binding domains with H X 1 E X 23-24 C X 2-4 C motifs, where X is any amino acid [4] . The histidine and cysteine residues coordinate Zn 2+ , while glutamic acid is thought to function as a proton shuttle during the deaminase reaction [5] . The single-domain A3A protein, the subject of this study, has multiple activities. A3A degrades foreign DNA introduced into human cells [6] , [7] and blocks replication of exogenous viruses such as human papilloma virus [8] , Rous sarcoma virus [9] , parvoviruses [10] , [11] and human T-lymphotropic virus type 1 (ref. 12 ). In addition, it strongly inhibits retrotransposition of LINE-1, Alu and LTR retroelements [10] , [13] , [14] , [15] , [16] , which cause insertional mutations. Unlike A3G (ref. 17 ), A3A is capable of deaminating 5-methylcytosine [18] , [19] , an epigenetic marker in genomic DNA, as well as inducing cell cycle arrest [20] and somatic hypermutation of nuclear and mitochondrial DNAs in a dynamic interplay between A3 editing and DNA catabolism [20] , [21] . How all these activities are regulated, however, is not fully understood, although Tribbles 3, a human protein, was recently reported to protect nuclear DNA from A3A-mediated deamination [22] . A3A is highly expressed in cells of the myeloid lineage, such as monocytes and macrophages, and its expression is upregulated by treatment with interferon-alpha [10] , [23] , [24] , [25] , [26] . Interestingly, silencing of A3A in monocytes is associated with increased susceptibility to human immunodeficiency virus (HIV)-1 infection, suggesting that the presence of A3A may be protective against HIV-1 (ref. 23 ). Recent studies indicate that endogenous A3A in macrophages restricts HIV-1 replication by reducing synthesis of viral DNA during reverse transcription [27] . This result is consistent with an independent observation that HIV-1 transcripts in interferon-alpha-treated infected macrophages seem to be edited predominantly by A3A (ref. 28 ). Although abundant information on the biological activities of the A3 proteins has been reported, only limited structural data are available. For example, the structure of the C-terminal domain (CTD) of A3G, which contains the catalytic centre for its deaminase activity [17] , [29] , [30] , was solved by nuclear magnetic resonance (NMR) [31] , [32] , [33] and X-ray crystallography [34] , [35] , but the structure of full-length A3G has been more elusive. While this manuscript was in preparation, the X-ray structure of another single-domain A3 protein, A3C, was reported [36] . Given human A3A’s function as an inhibitor of retroviruses and retroelements with significant effects on cellular activities, the availability of an atomic, three-dimensional structure clearly is of significant importance. Here we report the NMR solution structure of human A3A, define the interface that is critical for its interaction with single-stranded oligonucleotide substrates and characterize its catalytic activity. Detailed analysis of A3A binding to nucleic acids and real-time monitoring of the deamination reaction by NMR allow us to propose a mechanism for substrate selection and specificity. These studies provide the structural basis for a deeper understanding of A3A’s biological activities and broaden our knowledge of the molecular properties of the A3 proteins. Biochemical characterization of purified A3A To ensure that the purified, recombinant wild-type A3A (199 aa), (containing a C-terminal His 6 -tag (LEHHHHHH)), was enzymatically active, a uracil DNA glycosylase (UDG)-dependent gel-based deaminase assay was performed ( Fig. 1a ). The catalytic activity of this tagged protein was evaluated using a fluorescently labelled 40-nt ssDNA substrate, containing the TT C A deaminase recognition site, in the presence of increasing concentrations of protein, ranging from 20 to 1000, nM. Over 50% of the substrate was converted to the deaminated product with as little as 20 nM A3A, and complete conversion was seen with 200 nM A3A. These results demonstrate that the recombinant A3A protein is highly active as a cytidine deaminase. 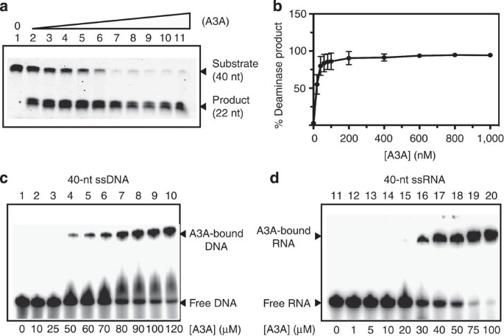Figure 1: Deaminase activity and ssDNA and ssRNA binding of A3A. (a) Deamination of a 40-nt ssDNA as a function of A3A concentration measured in a UDG-dependent assay. Reactions were performed as described in Methods with increasing concentrations of A3A. Lanes: 1, no A3A; 2, 20 nM; 3, 40 nM; 4, 60 nM; 5, 80 nM; 6, 100 nM; 7, 200 nM; 8, 400 nM; 9, 600 nM; 10, 800 nM; 11, 1000, nM, and relative amounts of substrate and product were assessed by gel electrophoresis. A representative gel (of three independent assays) was chosen for the figure. (b) Quantification of the relative amounts of deaminase product versus A3A concentration from gel analysis as shown in (a). The error bars represent the s.d. for three independent measurements. (c,d) Binding of A3A to 40-nt ssDNA (c) or 40-nt ssRNA (d) evaluated by electrophoretic mobility shift assay (EMSA; details in Methods). The positions of the A3A-bound as well as free DNA or RNA are indicated. A3A concentrations are listed under each lane. In each case, a representative gel (of five independent assays) was chosen for the figure. Figure 1: Deaminase activity and ssDNA and ssRNA binding of A3A. ( a ) Deamination of a 40-nt ssDNA as a function of A3A concentration measured in a UDG-dependent assay. Reactions were performed as described in Methods with increasing concentrations of A3A. Lanes: 1, no A3A; 2, 20 nM; 3, 40 nM; 4, 60 nM; 5, 80 nM; 6, 100 nM; 7, 200 nM; 8, 400 nM; 9, 600 nM; 10, 800 nM; 11, 1000, nM, and relative amounts of substrate and product were assessed by gel electrophoresis. A representative gel (of three independent assays) was chosen for the figure. ( b ) Quantification of the relative amounts of deaminase product versus A3A concentration from gel analysis as shown in ( a ). The error bars represent the s.d. for three independent measurements. ( c , d ) Binding of A3A to 40-nt ssDNA ( c ) or 40-nt ssRNA ( d ) evaluated by electrophoretic mobility shift assay (EMSA; details in Methods). The positions of the A3A-bound as well as free DNA or RNA are indicated. A3A concentrations are listed under each lane. In each case, a representative gel (of five independent assays) was chosen for the figure. Full size image Binding of A3A to ssDNA and ssRNA was evaluated in electrophoretic mobility shift assay experiments with 32 P-labelled 40-nt oligonucleotides and varying concentrations of A3A ( Fig. 1c ). Complexes are seen at A3A concentrations of ≥50 μM with ssDNA ( Fig. 1c , lane 4) and ≥20 μM with ssRNA ( Fig. 1d , lane 15). To achieve ~ 50% complexation, twofold more A3A (80 μM) was required for ssDNA ( Fig. 1c , lane 7), compared with ssRNA (40 μM) ( Fig. 1d , lane 17), suggesting that A3A has a somewhat higher binding affinity for ssRNA than that for ssDNA. Estimated K d values of ~ 80 μM for the A3A–ssDNA complex agree well with values derived from NMR titration data (see below). NMR sample preparation and behaviour in solution Full-length A3A was monomeric and soluble up to ∼ 0.2 mM at pH 6.5, 200 mM NaCl, and the 1 H– 15 N heteronuclear single quantum coherence (HSQC) spectrum exhibited well dispersed, narrow resonances ( Fig. 2 ). Nearly complete backbone and side-chain assignments were obtained using unlabelled, uniformly 15 N-, 13 C/ 15 N- and 2 H/ 13 C/ 15 N-labelled A3A with specific-protonations (see Methods ) for three different conditions: (1) ~ 0.2 mM A3A at pH 6.5, 200 mM NaCl ( Fig. 2 ); (2) ~ 0.2 mM A3A at pH 6.9; and (3) ~ 0.3 mM A3A at pH 8.1, all in 25 mM sodium phosphate buffer. As essentially identical nuclear Överhauser effect (NOE) patterns and chemical shifts were observed for the different conditions (only the amide resonances exhibited small, pH-dependent chemical shift differences), the structure was assumed to be unaffected by these different conditions. A mutant A3A, L63N/C64S/C171Q, was also used to help resolve ambiguous assignments (see Methods ). 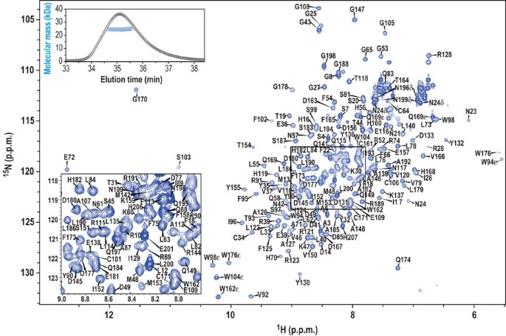Figure 2: A3A NMR assignments. 600 MHz1H–15N HSQC NMR spectrum of 0.17 mM13C/15N-labelled A3A in 25 mM sodium phosphate, 200 mM NaCl, pH 6.5, 25 °C. Assignments are indicated by residue name and number. An expansion of the boxed region is provided in the lower left corner. Size-exclusion chromatography/multi-angle light scattering data are shown in the inset in the upper left corner, with the elution profile shown with black circles and the estimated molecular masses across the peak with blue triangles. Figure 2: A3A NMR assignments. 600 MHz 1 H– 15 N HSQC NMR spectrum of 0.17 mM 13 C/ 15 N-labelled A3A in 25 mM sodium phosphate, 200 mM NaCl, pH 6.5, 25 °C. Assignments are indicated by residue name and number. An expansion of the boxed region is provided in the lower left corner. Size-exclusion chromatography/multi-angle light scattering data are shown in the inset in the upper left corner, with the elution profile shown with black circles and the estimated molecular masses across the peak with blue triangles. Full size image A3A structure The structure of full-length A3A was calculated on the basis of 3279 NMR-derived experimental constraints. The final model satisfies all experimental constraints, displays excellent covalent geometry and the 30-conformer ensemble exhibits atomic r.m.s. deviations of 0.60±0.05 and 1.18±0.05 Å with respect to the mean coordinate positions for the backbone (N, C α , C′) and all heavy atoms, respectively ( Table 1 ). A stereoview of the ensemble of conformers as well as a ribbon representation of the lowest energy structure from the ensemble are depicted in Fig. 3a , respectively. Table 1 Statistics for the final 30 conformer ensemble of A3A. 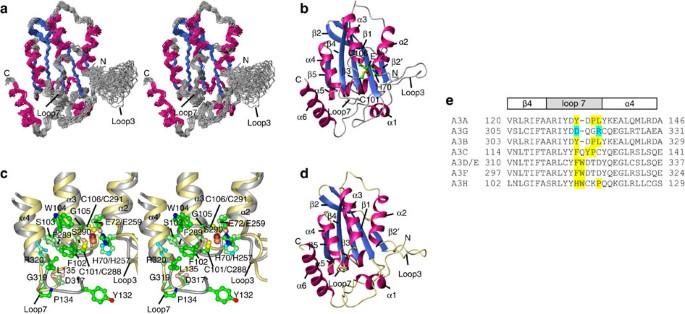Figure 3: A3A NMR solution structure. (a) Stereoview of the final 30 conformer ensemble (N, Cα, C′). Regions of helical and beta sheet structures are coloured hot pink and royal blue, respectively, and the remainder of the structure in grey. (b) Ribbon representation of the lowest energy structure of the ensemble, using the same colour scheme as in (a). Secondary structure elements are labelled and the active site residues (H70, E72, C101 and C106) and the Zn2+ion are shown in ball-and-stick representation with carbon, nitrogen, oxygen, sulphur and Zn atoms in green, blue, red, yellow and brown, respectively. (c) Stereoview of the superimposition of the active site regions of the current A3A NMR and the A3G-CTD (PDB: 3IR2) X-ray structures. The backbone traces of A3A and A3G-CTD are coloured grey and khaki, respectively. Side chains are shown in ball-and-stick representation with carbon, nitrogen, oxygen, sulphur and Zn atoms of A3A and A3G in green, blue, red, yellow and brown, and pale green, cyan, pink, yellow and orange, respectively. A3A residues are labelled in bold. (d) Ribbon representation of the A3G-CTD (A3G191-384-2K3A, PDB: 3IR2) X-ray structure35. (e) Amino-acid sequences of the loop 7 region in different A3 proteins. Large, hydrophobic residues are highlighted in yellow and the polar residues D317 and R320 in A3G are highlighted in cyan. Full size table Figure 3: A3A NMR solution structure. ( a ) Stereoview of the final 30 conformer ensemble (N, Cα, C′). Regions of helical and beta sheet structures are coloured hot pink and royal blue, respectively, and the remainder of the structure in grey. ( b ) Ribbon representation of the lowest energy structure of the ensemble, using the same colour scheme as in ( a ). Secondary structure elements are labelled and the active site residues (H70, E72, C101 and C106) and the Zn 2+ ion are shown in ball-and-stick representation with carbon, nitrogen, oxygen, sulphur and Zn atoms in green, blue, red, yellow and brown, respectively. ( c ) Stereoview of the superimposition of the active site regions of the current A3A NMR and the A3G-CTD (PDB: 3IR2) X-ray structures. The backbone traces of A3A and A3G-CTD are coloured grey and khaki, respectively. Side chains are shown in ball-and-stick representation with carbon, nitrogen, oxygen, sulphur and Zn atoms of A3A and A3G in green, blue, red, yellow and brown, and pale green, cyan, pink, yellow and orange, respectively. A3A residues are labelled in bold. ( d ) Ribbon representation of the A3G-CTD (A3G191-384-2K3A, PDB: 3IR2) X-ray structure [35] . ( e ) Amino-acid sequences of the loop 7 region in different A3 proteins. Large, hydrophobic residues are highlighted in yellow and the polar residues D317 and R320 in A3G are highlighted in cyan. Full size image Overall, the A3A structure consists of six helices surrounding a central β sheet of five strands ( Fig. 3a ), common to all APOBEC proteins whose structures are known; that is, A3G-CTD, A3C and A2 ( Supplementary Table S1 ). The structured region of A3A is limited to residues 10–194 ( Fig. 3a ), as very intense, sharp amide resonances, exhibiting random-coil chemical shifts ( Fig. 2 ), are present for the N-terminal nine (1–9) and final five (195–199) residues in the A3A sequence as well as the His 6 -tag residues, indicating a substantial degree of flexibility. In addition to the termini, the loop connecting β2' and α2 (loop 3, residues 57–70; Fig. 3a ) is also highly plastic and undergoes motions on an intermediate (μ-ms) timescale, as many amide resonances exhibit severe line broadening, and are of low intensity (Q58, N61, L62) or entirely missing (A59, Y67 and G68) in the 1 H– 15 N HSQC spectrum ( Fig. 2 ). This is suggestive of multiple conformations undergoing chemical exchange. Comparison with other APOBEC protein structures We carried out a detailed comparison of the present A3A solution structure with other available structures of APOBEC proteins ( Supplementary Table S1 ). Among these structures, the present A3A NMR structure is most similar to the X-ray structure of the A3G-CTD quintuple mutant (residues 191–384, PDB: 3IR2) [35] ( Fig. 3c ), exhibiting an average pairwise backbone atomic r.m.s. difference of 1.86 Å. The next closest structures are the X-ray structures of wild-type A3C, another single-domain human A3 protein (1–190, PDB: 3VOW) [36] , and wild-type A3G-CTD (residues 197–380, PDB: 3E1U/3IQS) [34] , both exhibiting average backbone r.m.s. differences of ~ 2.3–2.4 Å. The NMR solution structures of monomeric A2 proteins (murine A2, PDB: 2RPZ and a CS-HM Rosetta model for human A2 (ref. 37 )) are also similar to A3A (atomic r.m.s. differences of ~ 3.4 Å). In the previously solved A3G-CTD structures, some local differences were reported [31] , [32] , [33] , [34] . Our current A3A structure clearly possesses an interrupted β2 strand (β2-bulge-β2′; Fig. 3b and Supplementary Fig. S1 ), as well as an N-terminal α-helix (α1, residues 15–21). A more detailed comparison was carried out between the current A3A and the most similar A3G-CTD structures (A3G191-384-2K3A; Fig. 3c and Supplementary Table S1 ). We focused on the regions around the active site where the A3A and A3G sequences differ. A two amino-acid (W104 and G105) insertion, located between two Zn-coordinating cysteines (C101 and C106) in the active site of A3A, is the most prominent sequence change. Despite this insertion, the positions of the catalytic site residues H70 (H257 in A3G), E72 (E259), C101 (C288) and C106 (C291) are very similar in both structures ( Fig. 3c ). The insertion, however, distorts the N-terminal end of helix α3, with W104 bulging out, causing positioning of the backbone and/or side chain atoms of S103 and G105 in A3A equivalent to those of F289 and S290 in A3G. This structural adjustment places the hydrophobic F102 and W104 side chains at the protein surface, next to the active site. In contrast, A3G possesses only one hydrophobic residue (F289) in this region. Loop 7 is located near the active site ( Fig. 3 ), and its C-terminal half in A3G is known to have an important role in substrate selection (TC or CC) [38] . In A3A, loop 7 (127–135) adds additional hydrophobic residues (Y132, P134 and L135), whereas in A3G two of the equivalent residues (D317 and R320) are polar, and the proline is replaced by glycine, resulting in conformational differences between the A3A and A3G loop 7 ( Fig. 3c ). Note that among the human A3 proteins, the polar characteristic of this region is unique for A3G ( Fig. 3e ). A3A interacts with dCTP and dUTP Although A3A is a well-known cytidine deaminase, the determinants of substrate specificity (that is, preferential recognition of TC (refs 7 , 10 , 39 )) have not been characterized in detail. As an initial approach, we investigated binding of A3A to dCTP, several ssDNA oligonucleotide substrates and/or their dU-containing products by NMR. dUTP ( Fig. 4a ) and dCTP ( Fig. 4e ) binding was monitored by 1 H– 15 N HSQC spectroscopy, and affected regions were mapped onto the A3A structure (insets). Perturbations of amide resonances of the active site amino acids H70, E72, C101 and C106 as well as other surrounding ones (K30, L55, H56, N57, Q58, K60, N61, L63, C64, H70, A71, W98, S99 and Y132) were very similar, indicating that both the substrate and the product bind to the active site. Several of the amino acids whose resonances were affected reside in loop 3, with N61, L63 and C64 located distal to the active site, indicating that a remote conformational change was induced by dCTP/dUTP binding or that a particular preferred conformation was selected from the flexible ensemble in the substrate-free A3A state. Titration curves of selected perturbed resonances upon dCTP ( Fig. 4e ) and dUTP ( Fig. 4a ) binding were used to extract K d values of 536±72 μM and 578±115 μM, respectively ( Table 2 ). Note that as up to 30% of the dCTP was converted to dUTP during the titration, the value for dCTP should be regarded as an approximation. 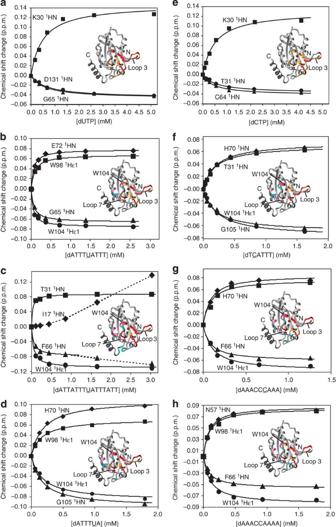Figure 4: Binding of A3A to mononucleotides and ssDNAs. Titration curves for representative HN resonances and binding site mapping (inset) for binding of dUTP (a), ATTTUATTT (b), ATTATTTUATTTATT (c), ATTTUA (d), dCTP (e), TCATTT (f), AAACCCAAA (g) and AAACCAAAA (h). A3A residues whose resonances exhibit large1H,15N-combined chemical shift changes upon nucleotide addition are coloured red (>0.050 p.p.m.) and orange (0.028–0.050 p.p.m.). Those only affected by ssDNA binding, but not by dCTP/dUTP, are shown in dark pink (>0.050 p.p.m.) and cyan (0.028–0.050 p.p.m.). All1H–15N HSQC spectra were recorded at 25°C using 25 mM sodium phosphate buffer, pH 6.9.1H,15N-combined chemical shift changes were calculated using, with ΔδHNand ΔδN, the1HN and15N chemical shift differences observed for A3A before and after adding ligands (~ 90% saturation). Figure 4: Binding of A3A to mononucleotides and ssDNAs. Titration curves for representative HN resonances and binding site mapping (inset) for binding of dUTP ( a ), ATTT U ATTT ( b ), ATTATTT U ATTTATT ( c ), ATTT U A ( d ), dCTP ( e ), T C ATTT ( f ), AAACC C AAA ( g ) and AAAC C AAAA ( h ). A3A residues whose resonances exhibit large 1 H, 15 N-combined chemical shift changes upon nucleotide addition are coloured red (>0.050 p.p.m.) and orange (0.028–0.050 p.p.m.). Those only affected by ssDNA binding, but not by dCTP/dUTP, are shown in dark pink (>0.050 p.p.m.) and cyan (0.028–0.050 p.p.m.). All 1 H– 15 N HSQC spectra were recorded at 25°C using 25 mM sodium phosphate buffer, pH 6.9. 1 H, 15 N-combined chemical shift changes were calculated using , with Δ δ HN and Δ δ N , the 1 HN and 15 N chemical shift differences observed for A3A before and after adding ligands (~ 90% saturation). Full size image Table 2 Dissociation and catalytic constants for A3A interaction with ss deoxymono- and deoxyoligonucleotides. * Full size table A3A binds ssDNA substrates via an extended surface The interaction of 5′-ATTT C ATTT-3′ (~ 0.1–3 mM) with A3A (~ 0.15 mM) under our NMR conditions resulted in conversion to 5′-ATTT U ATTT-3′ within <1 min, rendering it impossible to measure a true K d value for 5′-ATTT C ATTT-3′. However, given the similarity between dUTP and dCTP binding to A3A ( Fig. 4a versus Fig. 4e ), it seemed reasonable to assume that 5′-ATTT U ATTT-3′ and 5′-ATTT C ATTT-3′ would also have similar binding properties. The K d value for the ATTT U ATTT product was 58±8 μM ( Fig. 4b , Table 2 ), and its interaction surface on the A3A structure ( Fig. 4b , inset) covers a larger surface, extending beyond the catalytic site. This extended interface involves an area to the left side of the active site, opposite of loop 3 (where residues are coloured in hot pink (Δ δ >0.050 p.p.m.) or cyan (Δ δ between 0.028 and 0.050 p.p.m.) in the ribbon diagram). Interestingly, the two-residue insertion (W104/G105), unique to A3A, is part of the interface: the W104 backbone amide (Δ δ =0.122 p.p.m.) and the W104 ε1 side chain resonance (Δ δ =0.079 p.p.m. ), as well as the G105 (Δ δ =0.066 p.p.m.) and S103 (Δ δ =0.072 p.p.m.) amide resonances exhibit the largest perturbations. In addition, loop 7 and helix α4 are also part of the extended interface, as effects on the amide resonances of residues D133 (Δ δ =0.112 p.p.m. ), L135 (Δ δ =0.102 p.p.m.) and E138 (Δ δ =0.079 p.p.m.) were observed. Additional binding studies of A3A using a 15-nt oligonucleotide, 5′-ATTATTT U ATTTATT-3′ yielded essentially the same binding site ( Fig. 4c , inset) and affinity ( K d =57±11 μM; Fig. 4c , Table 2 ), as found with the 9-mer. Although smaller perturbations were observed for some additional resonances, these changes were non-saturable and most likely reflect non-specific binding (for example, the I17 resonance marked by a dashed line in Fig. 4c ). The non-specific binding site of the 15-mer oligonucleotide mapped onto the A3A structure involves residues 12–19 (α1), 36–37, 40–42 (β1), 44–49 (β2), 53–56 (β2′) and 179–186 (α6) ( Supplementary Fig. S2 ). To validate the binding data, the interaction of an A3A catalytic site mutant, E72Q, with a 15-nt substrate 5-′(ATTATTT C ATTTATT)-3′ was evaluated. The mutant exhibited the same affinity ( K d =55±11 μM, data not shown) as wild-type A3A with the 5′-ATTATTT U ATTTATT-3′ product, confirming that binding of substrate and product occurs with essentially identical affinities. Further titration experiments using smaller oligonucleotides (5′-ATTT( C/U )A-3′, Fig. 4d ; 5′-T C ATTT-3′, Fig. 4f ) delineated a binding site similar to the one observed with the nona-nucleotide. This implies that three nucleotides, (T C A), constitute the essential moiety for binding to A3A. The affinities of the hexanucleotides, however, were approximately threefold weaker ( K d ~ 190 μM) than the one measured for 5′-ATTT( C/U )ATTT-3′ ( K d =58±8 μM; Table 2 ), suggesting a stabilizing effect of the flanking nucleotides in the complex. Interaction of A3A with a 9-nt substrate, 5′-AAACC C AAA-3′, containing the A3G deaminase-specific recognition site [2] , maps to the same surface ( Fig. 4g , inset) as 5′-ATTT( C/U )ATTT-3′ ( Fig. 4b , inset). This suggests that both dT and dC at the −1 and −2 positions, that is, pyrimidine bases, can interact with the extended interface next to the catalytic site of A3A. However, slightly weaker binding ( K d =91±15 μM, Fig. 4g , Table 2 ) was observed for 5′-AAACC C AAA-3′ compared with 5′-ATTT C ATTT-3′. Replacement of the central CCC in 5′-AAACC C AAA-3′ by CCA (5′-AAAC C AAAA-3′, Fig. 4h ) or CAA (5′-AAA C AAAAA-3′, Table 2 ) resulted in identical ( K d =94±11 μM) or slightly weaker ( K d =161±19 μM) affinities, respectively. Structural model for A3A–ssDNA complexes Model structures of the A3A-oligonucleotide complexes were created by flexible docking [40] and selecting binding poses compatible with chemical shift perturbations (see Methods for details). Initial docking results for 5′-ATTT C ATTT-3′ and 5′-AAACC C AAA-3′ indicated that only the central region of the oligonucleotides interacts specifically with A3A, leaving the two ends free. Therefore, we only generated final structural models of A3A with the pentanucleotides 5′-TT C AT-3′ ( Fig. 5a ) and 5′-CC C AA-3′ ( Fig. 5b ). In the A3A/TT C AT complex model, the central reactive C occupies the deep pocket delineated by the active site and surrounding residues T31, N57, Q58, H70, E72, W98, C101, C106, D131 and the Zn 2+ ion. The thymidine (T −1 ) immediately preceding the C interacts with a surface formed by residues D133, P134, L135 (loop 7) and F102 (loop 5), whereas T −2 contacts residues F102, S103, W104, and G105 (loop 5), L135 (loop 7) and E138 (α4). The adenosine (A +1 ) at the 3′ side of the C interacts with residues D131, Y132 and D133 (loop 7). The 5-methyl groups of T −1 and T −2 are in close contact with several hydrophobic residues, for example, F102, W104 and L135, suggesting that this hydrophobic interaction may contribute to tighter binding of TT C A- compared with CC C A-containing ssDNA. The model for the A3A/CC C AA complex ( Fig. 5b ) is very similar to that of A3A/TT C AT ( Fig. 5a ), including the localization of the individual nucleotides. 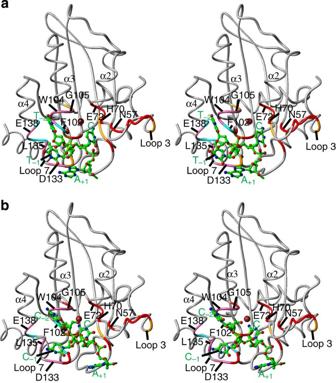Figure 5: Model of A3A complexed with TTCAT or CCCAA. Stereoviews of the A3A backbone structure and the 5-nt ssDNAs (TTCAT (a) and CCCAA (b)), as well as interacting residues (fromFig. 4borFig. 4g) in ball-and-stick representation, with carbon, nitrogen, oxygen, phosphorus and Zn atoms in green, blue, red, gold and brown, respectively. The 3′-end thymidine (a) and adenosine (b), which appear to be random, are omitted for clarity. Figure 5: Model of A3A complexed with TT C AT or CC C AA. Stereoviews of the A3A backbone structure and the 5-nt ssDNAs (TT C AT ( a ) and CC C AA ( b )), as well as interacting residues (from Fig. 4b or Fig. 4g ) in ball-and-stick representation, with carbon, nitrogen, oxygen, phosphorus and Zn atoms in green, blue, red, gold and brown, respectively. The 3′-end thymidine ( a ) and adenosine ( b ), which appear to be random, are omitted for clarity. Full size image Deamination by real-time NMR The A3A-catalyzed deamination reaction with several substrates was followed by two-dimensional (2D) 1 H– 13 C HSQC ( Fig. 6a ) or 1D 1 H ( Fig. 6b–d ) NMR. Using dCTP as the substrate, we determined that slow but measurable deaminase activity is present ( Fig. 6a ): at 25 °C, 5.2 mM dCTP was completely converted to dUTP by 170 μM A3A in ~ 50 h. Longer substrates, such as the 9-nt 5′-ATTT C ATTT-3′, were deaminated much more rapidly ( Fig. 6b ), and in such cases 1D 1 H NMR spectroscopy was used ( Fig. 6b inset). The 9-nt substrate (0.98 mM) was completely deaminated by 0.196 μM A3A in ~ 1.7 h, with an initial rate of ~ 0.8 mM h −1 . Other substrates, a 15-mer, 5′-ATTATTT C ATTTATT-3′, and two hexanucleotides, 5′-ATTT C A-3′ and 5′-T C ATTT-3′, ( Supplementary Fig. S3a–c , respectively) exhibited essentially identical rates to that observed with the nona-nucleotide. 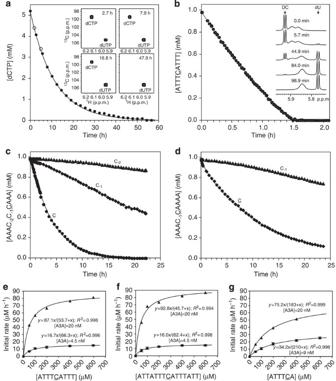Figure 6: A3A-catalyzed deamination of dCTP and several ssDNA substrates monitored by real-time NMR. Concentrations of dCTP (a), 9-nt ssDNA ATTTCATTT (b), AAAC−2C−1CAAA (c) and AAAC−1CAAAA (d) versus incubation time are provided. All concentrations of unreacted substrates (cytidine) and end products (uridine) were determined by measuring the intensities of the13C-5-1H resonances of cytosine and uracil in the 2D1H–13C HSQC spectra (a; 600 MHz) or the1H-5 resonances in 1D1H spectra (b–d; 900 MHz), as a function of time. The A3A concentration was 0.17 mM (a) or 0.197 μM (b–d). Best fit curves are shown by a solid line. Representative 2D1H–13C HSQC (a) or 1D1H NMR (b) spectra acquired at the indicated times are shown in the inset. (e–g) Kinetics of A3A-catalyzed deamination reactions for ATTTCATTT (e), ATTATTTCATTTATT (f) and ATTTCA (g); initial reaction rates (<5%) are plotted versus substrate concentrations. Reactions were monitored by 1D1H real-time NMR (900 MHz) at 25 °C in 25 mM sodium phosphate buffer, pH 6.9. Two different A3A concentrations were used: (eandf), 4.5 nM (circles) and 20 nM (triangles); (g), 9.0 nM (circles) and 20 nM (triangles). Two independent experiments were performed with 4.5 and 9 nM A3A and average values with s.d. are shown. Reactions with the higher A3A concentration (20 nM) resulted inKMandkcatvalues very similar to those obtained with low A3A concentrations (4.5 or 9 nM). Figure 6: A3A-catalyzed deamination of dCTP and several ssDNA substrates monitored by real-time NMR. Concentrations of dCTP ( a ), 9-nt ssDNA ATTT C ATTT ( b ), AAA C − 2 C − 1 C AAA ( c ) and AAA C − 1 C AAAA ( d ) versus incubation time are provided. All concentrations of unreacted substrates (cytidine) and end products (uridine) were determined by measuring the intensities of the 13 C-5- 1 H resonances of cytosine and uracil in the 2D 1 H– 13 C HSQC spectra ( a ; 600 MHz) or the 1 H-5 resonances in 1D 1 H spectra ( b – d ; 900 MHz), as a function of time. The A3A concentration was 0.17 mM ( a ) or 0.197 μM ( b – d ). Best fit curves are shown by a solid line. Representative 2D 1 H– 13 C HSQC ( a ) or 1D 1 H NMR ( b ) spectra acquired at the indicated times are shown in the inset. ( e – g ) Kinetics of A3A-catalyzed deamination reactions for ATTT C ATTT ( e ), ATTATTT C ATTTATT ( f ) and ATTT C A ( g ); initial reaction rates (<5%) are plotted versus substrate concentrations. Reactions were monitored by 1D 1 H real-time NMR (900 MHz) at 25 °C in 25 mM sodium phosphate buffer, pH 6.9. Two different A3A concentrations were used: ( e and f ), 4.5 nM (circles) and 20 nM (triangles); ( g ), 9.0 nM (circles) and 20 nM (triangles). Two independent experiments were performed with 4.5 and 9 nM A3A and average values with s.d. are shown. Reactions with the higher A3A concentration (20 nM) resulted in K M and k cat values very similar to those obtained with low A3A concentrations (4.5 or 9 nM). Full size image A3A and A3G purportedly possess a difference in substrate specificity [2] , [6] , [7] , [10] , [39] , [41] . To quantify A3A’s substrate specificity, we also assayed the deamination of an A3G-specific substrate, AAAC −2 C −1 C AAA, by A3A. Interestingly, all three cytidines were deaminated in a sequential 3′→5′ manner ( Fig. 6c ), with the third dC ( C ) converted with an initial rate of ~ 0.2 mM h −1 , only fourfold slower than the dC in the A3A-specific 5′-ATTT C ATTT-3′ substrate. When comparing substrates with varying numbers of cytosines, such as 5′-AAACC C AAA-3′ ( Fig. 6c ), 5′-AAAC C AAAA-3′ ( Fig. 6d ) and 5′-AAA C AAAAA-3′ ( Supplementary Fig. S3d ), deamination of the 3′ dC ( C ) was about two- to four-fold faster in 5′-AAACC C AAA-3′ than in the other two substrates, indicating a preference for two pyrimidine bases at the 5′ side of the reactive C . We also noted that the kinetics of the C→U conversions of C −1 and C −2 are much slower, quite distinct from that of C in the reaction with the AAAC −2 C −1 C AAA substrate. Similar behaviour was observed with AAAC −2 C −1 U AAA ( Supplementary Fig. S3e ), a substrate containing a uridine instead of the most reactive C. In contrast, when dC is followed by dA, and not by dU, for example, the C in 5′-AAAC −1 C AAA-3′ ( Fig. 6d ) and 5′-AAA C AAAAA-3′ ( Supplementary Fig. S3d ), the reaction proceeds readily, albeit somewhat slower than with AAAC −2 C −1 C AAA ( Fig. 6c ). Given our observation that dC and dU essentially possess the same A3A-binding affinities and interfaces, it seems reasonable to assume that once dC is converted to dU, competitive binding and inhibition occurs, slowing the deamination of C −1 and C −2 in AAAC −2 C −1 UAAA. Therefore, optimal substrates for A3A contain a cytidine preceded by two pyrimidine bases and followed by an adenine; that is, (T/C)(T/C) C A. Further studies were performed to determine the catalytic constants for A3A deaminase activity on single cytidine-containing substrates; that is, 5′-ATTT C ATTT-3′, 5′-ATTATTT C ATTTATT-3′, 5′-ATTT C A-3′, 5′-T C ATTT-3′ and 5′-AAA C AAAAA-3′. The kinetics of deamination revealed that all TCA-containing oligonucleotide substrates, regardless of length, exhibited identical turnover rates ( k cat ~ 60–70 min −1 ; Table 2 , Fig. 6e–g ). The hexanucleotides, however, displayed an approximately threefold lower apparent second-order rate constant ( k cat / K M ~ 5 × 10 3 M −1 s −1 ) than the one measured for the 9-nt and 15-nt substrates ( k cat / K M ~ 1.8 × 10 4 M −1 s −1 ), caused mainly by an increase in K M . For all A3A substrates, K M and K d values were very similar. A large reduction (~ 40-fold) of k cat / K M was seen only with a substrate that is lacking pyrimidine bases at the 5′ side of the reactive C ; that is, 5′-AAA C AAAAA-3′, caused by a large (13-fold) reduction in k cat and a small (approximately threefold) increase in K M (less-favourable binding), highlighting the importance of a pyrimidine base at the 5′ side. Collectively, the data in Fig. 6 demonstrate that the nucleotide context surrounding the reactive C is a major determinant of enzymatic activity. Here we present the NMR solution structure of human A3A as well as a detailed analysis of its nucleic acid interaction surface, providing new insights into substrate selection and binding. The A3A NMR structure very closely resembles the A3G-CTD and A3C X-ray structures [31] , [32] , [33] , [34] , [35] , [36] ( Supplementary Table S1 ) and not surprisingly, there are also similarities between the activities of A3A and the A3G-CTD. Using NMR, we show that A3A binds TTCA- or CCCA-containing single-stranded oligonucleotides (≥9 nt) with K d values ranging from 50–100 μM ( Table 2 ), in excellent agreement with binding affinity data (~ 80 μM) estimated from electrophoretic mobility shift assay ( Fig. 1c ) and with fluorescence depolarization results obtained by Love et al . [39] Intriguingly, A3A binds ssDNA much more weakly (~ 1000-fold) than A3G, for which K d values ranging from 50 to 240 nM have been reported [17] , [39] , [42] , [43] , [44] . However, like A3A, K d values (200–450 μM) were obtained for the single-domain A3G-CTD protein [31] , [32] , implying that the tighter binding of full-length A3G is associated with its double domain structure. Indeed, the A3G-N-terminal domain contains numerous positively charged amino acids that contribute to high efficiency binding to ssDNA [17] , [29] , whereas both A3A and the A3G-CTD are slightly acidic and are unable to interact in this manner. Importantly, titration of A3A with diverse ssDNA substrates by NMR made it possible to distinguish specific binding from non-specific binding ( Fig. 4c ). Our results showed that A3A can bind both TT C A- and CC C A-containing oligonucleotides, using the same five A3A contacts, namely the active site, loop 3, loop 5 including the exposed dipeptide W104-G105, loop 7 and helix α4. Surprisingly, although the W104NεH side chain resonance experiences the largest chemical shift changes upon substrate binding ( Fig. 4 ), W104 mutations do not seem to influence or abrogate A3A’s catalytic activity [16] , [18] . Note that A3A oligonucleotide-binding regions are highly localized and clustered around the active site, in stark contrast to results in the two studies that mapped ssDNA binding to A3G-CTD (refs 31 , 32 ). Interestingly, our A3A–ssDNA complex model ( Fig. 5 ) suggests that the DNA bends to insert the reactive cytidine into the active site, permitting only the immediate neighbouring (−1, −2 and +1) nucleotides to interact locally near the catalytic site. Interestingly, there are reports of RNA bending in the crystal structure of a transfer RNA adenosine deaminase/RNA complex [45] and DNA contraction during A3G scanning of the ssDNA substrate [46] . NMR real-time kinetic data for the deamination reaction of A3A using 5′-ATTT C ATTT-3′ and 5′-ATTATTT C ATTT-3′ as substrates yielded values of k cat ~ 70 min −1 and K M ~ 60 μM, which differ from the values ( k cat ~ 15 min −1 and K M ~ 230 nM) obtained using a 43-nt TT C T-containing ssDNA [18] . These differences may be related to variations in the ssDNA sequences and experimental conditions. Interestingly, Carpenter et al . reported that A3A is a stronger (~ 200-fold) deaminase than full-length A3G (ref. 18 ). Indeed, although similar amounts of deaminase product were observed in the NMR deamination assays described here for A3A ( Fig. 6b ) and for A3G-CTD in Furukawa et al . [32] , the amount of A3A used was 1000-fold less than the amount of A3G-CTD. The fact that A3A also deaminates the most 3′ dC ( C ) in 5′-AAACC C AAA-3′ (thought to be an A3G-specific substrate [2] ) with only an approximate fivefold reduction in k cat / K M , compared with TTCA-containing 9-nt and 15-nt oligonucleotides ( Table 2 ) appears puzzling at first. However, these results are in agreement with the deaminase specificity observed for A3A in cell-based assays. For example, in an investigation of foreign DNA restriction in human primary cells, A3A preferentially deaminated T C and C C sequences in the green fluorescent protein gene of the transfected plasmid DNA (ref. 6 ). In addition, a strong bias for deamination of T C (~ 50–70%) and C C (~ 15–25%) dinucleotide sequences was detected in nascent HIV-1 complementary DNAs isolated from infected macrophages [28] and in an in vitro HIV-1 model replication assay, performed using purified A3A protein [39] . Furthermore, a preference for T C and C C substrate recognition sites was also observed for A3A editing of human T-lymphotropic virus type 1 (ref. 12 ). Thus, A3A’s active site possesses the flexibility to accommodate and deaminate dC residues ( C ) in both T C and C C dinucleotides. Interestingly, in a study by Shinohara et al . [7] , it was shown that A3A mediates genomic DNA editing in human cells, but no editing site preference was detected. In contrast, Suspène et al . [21] found that A3A preferentially deaminates cytidines in T C and C C dinucleotides in genomic DNA, when cells are exposed to UDG inhibitor. APOBEC-mediated genomic DNA mutations have been implicated in carcinogenesis [47] and, for example, A3B was shown to be a source of DNA mutations in breast cancer [48] . These observations suggest that the strong mutagenic potential of A3A might be detrimental to the stability of the human genome. Thus, the dual function of A3A as a host restriction factor and as a DNA mutator that can potentially act on genomic DNA, an activity that may be associated with malignancies, suggests that A3A can act as a ‘double-edged sword’. The high resolution NMR structure of A3A presented here is a first step in aiding future structure-function studies for addressing these seemingly diverse A3A functions. Furthermore, the addition of the A3A structure to the still limited list of currently known APOBEC structures contributes to efforts towards elucidating the molecular mechanisms of the innate immune response. Protein expression and purification Wild-type (Accession number NM_145699), E72Q and L63N/C64S/C171Q mutant synthetic A3A genes with a C-terminal His 6 -tag (LEHHHHHH) were inserted into the Nde I– Xho I site of the pET21 plasmid (Novagen) for expression in Escherichia coli Rosetta 2 (DE3). Uniform 15 N- and 13 C-labelling of the proteins was carried out by growth in modified minimal medium at 18 °C, using 15 NH 4 Cl and 13 C 6 -glucose as the sole nitrogen and carbon sources, respectively. Uniform 2 H-, 15 N- and 13 C-labelling of the proteins was achieved using 2 H 2 O, 15 NH 4 Cl and 13 C 6 / 2 H 7 -glucose as deuterium, nitrogen and carbon sources, respectively, with two different selective protonation of the side chains of (1) Tyr/Phe/Ile residues and (2) Tyr/Phe/Trp/Ile/Val/Leu residues, by adding 0.10–0.15 mg of 13 C/ 15 N-tyrosine, -phenylalanine and -isoleucine (for sample 1), and 13 C/ 15 N-tyrosine and -phenylalanine, unlabelled tryptophan, 2-keto-butyrate (1,2,3,4- 13 C, 98%; 3,3'- 2 H, 98%, CIL, Andover, MA, USA) and 2-keto-3-methyl-butyrate (1,2,3,4- 13 C, 99%; 3,4,4',4''- 2 H, 98%, CIL; for sample 2), respectively. These chemicals were added to the culture 1 h before induction with 0.4 mM isopropyl-1-thio-β-D-galactopyranoside (total induction time=16 h). Proteins were purified over a 5-ml Hi-Trap His column (GE Healthcare) and Hi-Load Superdex 200 (1.6 cm × 60 cm) column, equilibrated in buffer containing 25 mM Tris–HCl (pH 7.5), 50 mM NaCl, 5% glycerol, 2 mM dithiothreitol (DTT) and 0.02% NaN 3 . Fractions containing A3A were further purified over an 8-ml MONO-Q column (GE Healthcare) in 25 mM Tris-HCl buffer (pH 8.5), 5% glycerol, 2 mM DTT and 0.02% sodium azide, employing a linear gradient of 0–1 M NaCl. The final A3A preparations were >99% pure, as estimated by SDS–polyacrylamide gel electrophoresis. The molecular mass of the A3A proteins were confirmed by LC-ESI-TOF mass spectrometry (Bruker Daltonics, Billerica, MA, USA). Multi-angle light scattering Size-exclusion chromatography/multi-angle light scattering data were obtained at room temperature using an analytical Superdex 200 (S200) column with in-line multi-angle light-scattering refractive index (Wyatt Technology, Inc., Santa Barbara, CA, USA) and ultraviolet (Agilent Technologies, Santa Clara, CA) detectors. One hundred microlitres of 78.4 μM A3A were applied to the S200 column pre-equilibrated and eluted with 25 mM sodium phosphate buffer (pH 6.5), 200 mM NaCl, 0.02% sodium azide and 1 mM DTT at a flow rate of 0.5 ml min −1 . Deaminase assay using fluorescent-tagged ssDNA substrates Deaminase assay conditions were adapted from Iwatani et al . [17] Forty microlitres reactions, containing 180 nM of a 40-nt ssDNA (JL913, 5′-ATT ATT ATT ATT ATT ATT ATT T C A TTT ATT TAT TTA TTT A-3′), labelled at its 5′ end with Alexa Fluor 488, (Integrated DNA Technologies (IDT, Coralville, IA, USA) and varying amounts of A3A in 10 mM Tris–HCl buffer, pH 8.0, 50 mM NaCl, 1 mM DTT, 1 mM EDTA, pH 8.0, and 10 units of E. coli UDG (New England BioLabs) were incubated at 37 ° C for 1 h. The reaction was stopped by incubation with Proteinase K (40 μg, Ambion) at 65 °C for 20 min, followed by sequential addition of 10 μl of 1 N NaOH for 15 min at 37 ° C and 10 μl of 1 N HCl. Ten microlitres aliquots of the final mixture were subjected to electrophoresis in a 10% denaturing polyacrylamide gel. Gels were scanned in fluorescence mode on a Typhoon 9400 Imager and the data were quantified using ImageQuant software (GE Healthcare). Electrophoretic mobility shift assay Ten microlitres reactions, containing varying amounts of A3A, 20 nM of a 5′ 32 P-labelled 40-nt ssDNA (JL895, identical sequence to JL913 but without the Alexa Fluor 488 label; Lofstrand Labs Ltd, Gaithersburg, MD, USA) or 40-nt ssRNA (JL931, identical sequence to JL895, except that U was substituted for T; IDT), were incubated with 4 U SUPERase IN (Ambion) at 37 °C for 10 min in 50 mM Tris–HCl buffer, pH 7.0, 100 mM NaCl, 1 mM DTT, 1% Ficoll-400 and 2.5 mM EDTA. Aliquots from each reaction were loaded onto an 8% native polyacrylamide gel in 40 mM Tris-acetate buffer, pH 8.4, 1 mM EDTA and 5% glycerol. One microlitre DNA Loading Gel Solution (Quality Biological, Inc.), containing bromphenol blue and xylene cyanol, was added to a control sample without A3A. Gels were run at 4 °C (5 mA) until the bromphenol blue dye had migrated ~ 2/3 through the gel. Radioactive products were detected with a Typhoon 9400 Imager and were quantified using ImageQuant software. NMR spectroscopy All NMR spectra for the structure determination of A3A were recorded at 25 °C on Bruker AVANCE900, AVANCE800, AVANCE700 and AVANCE600 spectrometers, equipped with 5 mm triple resonance, Z-axis gradient cryoprobes. The NMR samples contained unlabelled, 13 C/ 15 N- or 2 H/ 13 C/ 15 N-labelled A3A with two types of selective protonations (see above). At pH 6.9 and 8.1, A3A showed higher solubility (~ 0.5 and ~ 1 mM, respectively) than that at pH 6.5 (~ 0.2 mM). However, at these higher protein concentrations, soluble aggregation occurred, as evidenced by severe line broadening. We therefore performed all of our NMR experiments at concentrations of ~ 0.2–0.3 mM. The sample temperature in the spectrometer was calibrated with 100% methanol. Backbone and side chain resonance assignments were carried out using 2D 1 H– 15 N HSQC, 1 H– 13 C HSQC and nuclear Överhauser enhancement spectroscopy (NOESY) and three-dimensional (3D) HNCACB, HN(CO)CACB, HNCA, HN(CO)CA and HCCH-total correlation spectroscopy experiments [49] . Distance constraints were derived from 3D simultaneous 13 C- and 15 N-edited NOESY (ref. 50 ) and 2D NOESY experiments. All NOESY spectra were acquired at 800 or 900 MHz, using a mixing time of 100 ms (non-perdeuterated samples) or 150 ms (perdeuterated samples). Spectra were processed with TOPSPIN 2.1 (Bruker) and NMRPipe [51] , and analyzed using SPARKY3 (version 3.113; T.D. Goddard and D.G. Kneller, University of California, San Francisco) and NMRView J (version 8.0.3) [52] . NMR structure calculation All NOE cross peaks were assigned from the 3D and 2D NOESY spectra using the SPARKY3 assignment tool. Structure calculations were performed for A3A residues 1–199, using the anneal.py protocol in XPLOR-NIH (ref. 53 ). An iterative approach with extensive, manual cross-checking of all distance constraints against the NOESY data and the generated structures was employed. The final number of the NMR-derived constraints were 3279, with 2827 NOE distances, 152 H-bond distances identified from NOE patterns for helices and β-sheets, and 300 φ and ψ backbone torsion angles from TALOS calculations [54] . In addition, a Zn 2+ ion was added at a late stage in the calculations to coordinate with H70, C101 and C106 (refs 31 , 32 ) using constraints based on the X-ray structures of A3G-CTD (refs 34 , 35 ). Five hundred and twelve structures were generated and the 30 lowest energy structures were selected and analyzed using PROCHECK-NMR (ref. 55 ) ( Table 1 ). All structure figures were generated with MOLMOL (ref. 56 ). A3A nucleotide-binding site mapping and titration by NMR To monitor nucleotide binding to A3A, aliquots of 14–100 mM mono- or oligodeoxynucleotide stock solutions were added to 0.10–0.18 mM 13 C/ 15 N-labelled A3A. 100 mM dCTP and dUTP stock solutions were purchased from Promega (Madison, WI, USA) and HPLC-purified DNA oligonucleotides were obtained from IDT or Midland Co. (Midland, TX, USA). A series of 2D 1 H– 15 N HSQC titration spectra were acquired and binding isotherms were obtained by plotting 1 HN proton chemical shift change versus nucleotide concentrations for 5–8 unambiguously traceable amide resonances. Dissociation constants were calculated by non-linear best fitting of the isotherms using KaleidaGraph (Synergy Software, Reading, PA, USA), and values for 5–8 resonances were averaged. Real-time studies of A3A-catalyzed deamination A series of 2D 1 H– 13 C HSQC and/or 1D 1 H NMR spectra were acquired as a function of time, after addition of A3A to solutions of mono- or oligodeoxynucleotide. Concentrations of A3A and deoxynucleotides for the different samples are provided in the figure captions. The intensities of well-resolved 13 C-5- 1 H resonances (volumes in 2D 1 H– 13 C HSQC spectra) and/or 1 H-5 resonances (integrals in 1D 1 H spectra) of cytosine and uracil were used for quantification. Real-time monitoring of the A3A-catalyzed deamination reaction by NMR permitted the extraction of initial (<5% dC→dU conversion) rates for a series of substrate concentrations (50, 100, 200, 400 and 600 μM). k cat (V max /[A3A]) and K M values were obtained using the Michaelis–Menten module in Kaleidagraph. Molecular docking Structures of 5′-TT C AT-3′, 5′-CC C AA-3′, 5′-ATTT C ATTT-3′ and 5′-AAACC C AAA-3′ ssDNAs were generated by MacroMoleculeBuilder (version 2.8) [57] . The oligonucleotide and A3A NMR structures were converted to a mol2 file format using the Hermes programme (version 1.4) and standard Tripos atom and bond types. Docking was performed with the flexible docking programme GOLD version 5.1 ( [40] ), in combination with the Chemscore scoring function [58] . The Zn 2+ ion was chosen as the centre point in the docking and the radius was set to 20 Å. For each nucleotide, five independent docking runs into the five lowest energy NMR structures of A3A, each producing fifty binding poses, were performed using a population of 100 ligands, with a maximal number of genetic algorithm operations dependent on ligand size: 50,000 for 5′-TT C AT-3′ and 5′-CC C AA-3′, and 150,000 for 5′-ATTT C ATTT-3′ and 5′-AAACC C AAA-3′. Docking poses (1250) for the pentanucleotides were subjected to a two-step selection process utilizing the NMR data. In the first step, complexes were discarded if the oligonucleotide engaged in contacts with residues that did not exhibit experimental chemical shift changes. In the second step, structures were selected that exhibited good agreement with the NMR binding-site mapping data, taking the size of the chemical shift changes and the scoring value of the binding pose into account. The final structural models for A3A, complexed with 5′-TT C AT-3′ ( Fig. 5a ) and 5′-CC C AA-3′ ( Fig. 5b ), represent ~ 80% of all the structures that result from the selection process. Accession codes: The A3A atomic coordinates and NMR constraints have been deposited in the RCSB Protein Data Bank under accession code 2m65 , and the NMR chemical shift data have been deposited in the Biological Magnetic Resonance Bank under accession code 19108. How to cite this article: Byeon, I.-J. L. et al . NMR structure of human restriction factor APOBEC3A reveals substrate binding and enzyme specificity. Nat. Commun. 4:1890 doi: 10.1038/ncomms2883 (2013).